Gender identification of the Mesozoic birdConfuciusornis sanctus Hundreds of specimens of the beaked bird Confuciusornis sanctus have been recovered from Early Cretaceous lake deposits of northeastern China. These birds show remarkable variation in size and plumage, with some displaying two long, central ornamental rectrices (tail feathers) and others lacking them altogether. Although, traditionally specimens with ornamental rectrices were interpreted as males and those without them as females, this supposed sexual dimorphism has remained unconfirmed. Here we report on the discovery of medullary bone, a tissue unique to reproductively active female birds, in a specimen of C. sanctus (DNHM-D1874) lacking these feathers. Our discovery constitutes the first case of gender identification in a Mesozoic bird, and it provides undisputed evidence that individuals of C. sanctus without ornamental rectrices are females. By permitting gender identification in C. sanctus , our results provide insight into the onset of sexual maturity and attainment of adult body size of this and other early birds. Confuciusornis sanctus [1] is the most abundant species of the diverse fossil avifauna from the Early Cretaceous Jehol Group of northeastern China. A complete, articulated specimen of this early bird, DNHM-D1874 (Dalian Natural History Museum, China), preserves distinctive feathers around the body, but does not display any central ornamental rectrices associated with its well-preserved caudal region ( Fig. 1a ). The femoral dimensions (52 mm) suggest that DNHM-D1874 falls within the high end of the size range known for C. sanctus [2] . 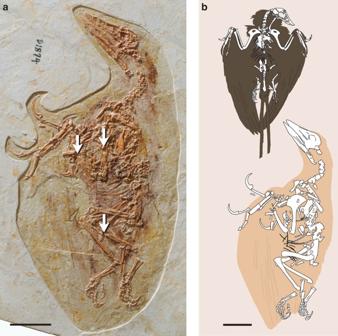Figure 1: Photograph and interpretive drawing of DNHM-D1874. (a) Arrows indicate the location of histological samples. (b) Drawing of DNHM-D1874 (below) compared with one of the smallest known specimens ofC. sanctusshowing ornamental rectrices (above) (GMV-2131, Geological Museum of China, Beijing). Scale bars equal 5 cm. Figure 1: Photograph and interpretive drawing of DNHM-D1874. ( a ) Arrows indicate the location of histological samples. ( b ) Drawing of DNHM-D1874 (below) compared with one of the smallest known specimens of C. sanctus showing ornamental rectrices (above) (GMV-2131, Geological Museum of China, Beijing). Scale bars equal 5 cm. Full size image Studies of bone histology are known to provide valuable insight pertaining to growth dynamics and biology of extinct animals [3] , [4] , [5] , [6] , [7] , [8] . The left humerus, tibia and ulna of DNHM-D1874 were therefore sampled for histological analyses. Our histological study detected the presence of medullary bone, thus indentifying DNHM-D1874 as a reproductively active female. Such discovery indicates that individuals of C. sanctus lacking ornamental rectrices are females. Framed within the context of the size distribution characteristic of this species, the discovery of medullary bone in DNHM-D1874 also indicates that C. sanctus , and other early birds, matured sexually well before reaching skeletal maturation. Histological analysis Examination of thin sections of the humerus reveals three distinct layers in the compacta: Outermost is the more slowly formed lamellar bone of the outer circumferential layer, wherein at least two lines of arrested growth are visible; internal to this is the reticular fibro-lamellar bone tissue formed during early ontogeny; and below this is a thick inner circumferential layer ( Fig. 2a ). Internal to the inner circumferential layer and extending from the endosteal margin into the medullary cavity is a layer of medullary bone (Mb) ( Fig. 2 ). This well vascularized, endosteally formed tissue characteristically has a cancellous or spongy texture and consists of woven bone [9] , [10] , [11] , [12] , [13] . Endosteal deposits are sometimes caused by disease (for example, avian osteopetrosis) and in such cases they are usually accompanied by bony periosteal outgrowths [13] . In DNHM-D1874, the periosteal surface of the humerus (and other bones in the skeleton) does not have any reactive deposits, which supports our conclusion that the endosteally derived tissue is not pathologic in origin. Furthermore, although the partial bone wall of DNHM-D1874 might suggest that the bone within the medullary cavity corresponds to displaced pieces of the compact bone wall, differences in the texture (spongy versus compact) and location (medullary bone spicules are outgrowths of the endosteal surface) ( Fig. 2b ) precludes them from being mistaken for one another. 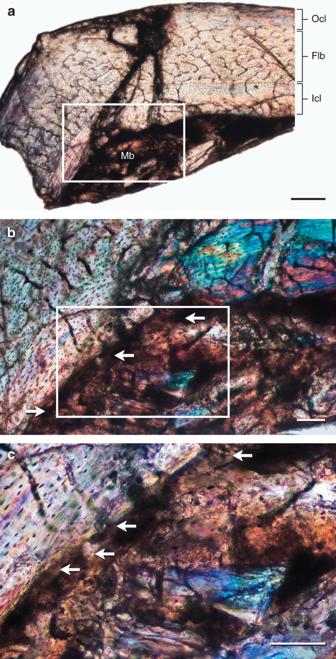Figure 2: Bone microstructure of DNHM-D1874. (a) Low magnification of a transverse section of the humerus of DNHM-D1874 showing the triple-layered compact bone wall with outer circumferencial layer (Ocl), fibro-lamellar bone (Flb) and inner circumferencial layer (Icl), and the medullary bone (Mb) within the medullary cavity. (b) Higher magnification (white box ina) showing the spongy texture of the medullary bone and the infrequent direct connections to the endosteal margin of the bone wall (white arrows). (c) Higher magnification of framed region inb; white arrows indicate the bony outgrowths of medullary bone from the endosteal region of the Icl. Scale bars, 300 μm (a) and 100 μm (b,c). Figure 2: Bone microstructure of DNHM-D1874. ( a ) Low magnification of a transverse section of the humerus of DNHM-D1874 showing the triple-layered compact bone wall with outer circumferencial layer (Ocl), fibro-lamellar bone (Flb) and inner circumferencial layer (Icl), and the medullary bone (Mb) within the medullary cavity. ( b ) Higher magnification (white box in a ) showing the spongy texture of the medullary bone and the infrequent direct connections to the endosteal margin of the bone wall (white arrows). ( c ) Higher magnification of framed region in b ; white arrows indicate the bony outgrowths of medullary bone from the endosteal region of the Icl. Scale bars, 300 μm ( a ) and 100 μm ( b , c ). Full size image Several studies have shown that the deposition of avian medullary bone is directly linked to the maturation of the ovarian follicles before egg laying, and that it acts as a calcium reservoir for the production of the calcareous eggshell [9] , [10] , [11] , [12] , [13] , [14] , [15] . The deposition of medullary bone is considered to be an adaptation to compensate for the thin-walled bones of birds, from which extensive bone resorption leads to brittleness and susceptibility to fractures [11] , [14] , [15] . Thus, our discovery of medullary bone directly indicates that DNHM-D1874, a specimen lacking ornamental rectrices, is a reproductive female. The fact that the medullary bone of DNHM-D1874 appears to be in a resorptive state in the humerus and only traces remain in the ulna, suggests that eggshell calcification had occurred and that an indeterminate number of eggs had been laid before death. The discovery of medullary bone in DNHM-D1874 sheds light on the biological significance of the variation in the tail plumage of C. sanctus . Although most researchers considered such variation as expressions of sexual dimorphism [16] , [17] , [18] , [19] , whether it was instead the result of moulting or some other biological manifestations could not be ruled out [1] . In addition, previous large-sample morphometric studies failed to provide definitive support for the presence of rectricial sexual dimorphism [2] . The current unequivocal identification of DNHM-D1874 as a female supports the hypothesis that individuals of C. sanctus without central ornamental rectrices are females and those displaying them are males. This interpretation is congruent with absence of medullary bone in three sampled specimens that distinctly present a pair of central ornamental rectrices ( Methods ). The detailed bone microstructure of both the humerus and the ulna indicates that DNHM-D1874 had passed its most rapid (juvenile) phase of growth [20] and that its growth rate had dramatically slowed down. Size comparisons with other specimens in our sample indicate that DNHM-D1874 was substantially smaller than the largest known specimens of C. sanctus ( Fig. 3 ). The presence of multiple lines of arrested growth—structures consistently interpreted as annual pauses in growth [21] , [22] , [23] , [24] —directly indicates that skeletal maturity occurred over several years, and that DNHM-D1874 was in its third year of growth. Ornamental rectrices in specimens with femora that are 69% the size of DNHM-D1874 (and 60% the largest specimen recorded by Marugán-Lobon et al. [2] ) ( Fig. 3 ) indicate that such dimorphism in C. sanctus developed well before skeletal maturity—our mass estimates (see Methods ) indicate that the smallest, sexually mature specimens had ∼ 23% the mass of the largest specimens in our sample ( Fig. 3 ). This further implies that unlike modern birds and similar to their nonavian ancestors [24] , [25] sexual maturity occurred well before skeletal maturation. Histological studies of other premodern birds have suggested that the extant condition of generally attaining adult body size within the first year of life, evolved late in the history of birds [6] , [21] , [22] . Our findings suggest that in addition, early birds also attained sexual maturity much earlier in ontogeny than their modern relatives. 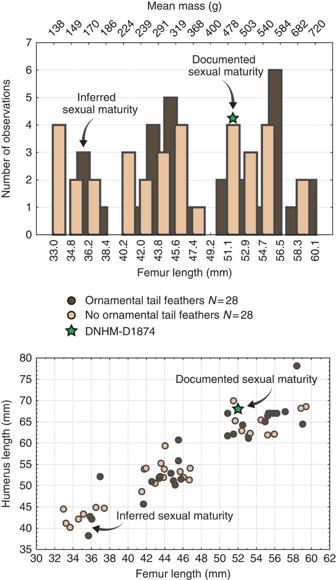Figure 3: Size distribution inC. sanctus. Frequency distribution of the lengths of the femur and scatterplot of the femur versus humerus. Plotted specimens include only those in which the presence or absence of ornamental rectrices was determined according to the criteria described underMethods.N=29 (DNHM-D1874 included) without ornamental rectrices andN=28 with ornamental rectrices. The discovery of medullary bone in DNHM-D1874 directly infers sexual maturity in comparably sized specimens. The presence of ornamental rectrices in much smaller specimens is used as a proxy for sexual maturity. Figure 3: Size distribution in C. sanctus . Frequency distribution of the lengths of the femur and scatterplot of the femur versus humerus. Plotted specimens include only those in which the presence or absence of ornamental rectrices was determined according to the criteria described under Methods . N =29 (DNHM-D1874 included) without ornamental rectrices and N =28 with ornamental rectrices. The discovery of medullary bone in DNHM-D1874 directly infers sexual maturity in comparably sized specimens. The presence of ornamental rectrices in much smaller specimens is used as a proxy for sexual maturity. Full size image Sampling and thin section preparation This study is part of a multi-year project aimed at understanding the life history of C. sanctus . In the course of this research, hundreds of specimens were photographed and measured for the purpose of morphological and morphometric analyses [1] , [2] . Plumage variation (that is, presence or absence of long ornamental rectrices) was determined upon close examination of the caudal region of each specimen: long ornamental rectrices were considered absent only on specimens in which the outline of the plumage around the pygostyle was well preserved, offering strong evidence that the absence of these feathers was not the result of taphonomy. Multiple bones (humerus, radius, ulna, tibia and femur) of 11 individuals were sampled for histological analyses. In three specimens, ornamental rectrices were clearly visible, whereas in six others they were not present, and in two specimens the caudal regions were not well preserved. Of the six specimens without ornamental rectrices, only DNHM-D1874 appeared to be reproductively active (that is, breeding) at the time of death, and thus preserved medullary bone tissue. It should be noted that our histological analyses of the three specimens with ornamental rectrices did not find evidence of medullary bone. The sampled bone pieces of the left humerus, tibia and ulna of DNHM-D1874 were embedded in Struers epoxy, and thin sectioned using standard histological methods [10] . Four thin sections of the humerus, and two thin sections of the ulna and tibia were prepared at the University of Cape Town in South Africa. The sections were studied under a biological petrographic microscope (Nikon Eclipse E200). The bone histology of the humerus and ulna were well preserved, but the tibial sample was incomplete and unsuitable for histological analyses. Both the humerus and the ulna preserved medullary bone around the edges of the medullary cavity, although the humeral sample was better preserved. Photomicrographs were taken using a Nikon DS-Fi1 digital camera and the imaging program NIS Elements version 3.2. Body mass calculation Body mass estimates (in g) in Fig. 3 correspond to allometric mean values calculated on the basis of the length of the femur (in mm). These mean values were calculated from the body mass estimates derived from the equations of Maloiy et al. [26] and Alexander [27] , as listed by Hone et al. , [28] and the equation of Peters and Peters [29] , which was modified from that of Prange et al. [30] ( Table 1 ). Table 1 Equations used to calculate the mean values for the mass of the specimens plotted in Fig. 3 . Full size table How to cite this article: Chinsamy, A. et al. Gender identification of the mesozoic bird Confuciusornis sanctus . Nat. Commun. 4:1381 doi: 10.1038/ncomms2377 (2013).